Elucidating the charge carrier separation and working mechanism of CH3NH3PbI3−xClxperovskite solar cells Developments in organic–inorganic lead halide-based perovskite solar cells have been meteoric over the last 2 years, with small-area efficiencies surpassing 15%. We address the fundamental issue of how these cells work by applying a scanning electron microscopy-based technique to cell cross-sections. By mapping the variation in efficiency of charge separation and collection in the cross-sections, we show the presence of two prime high efficiency locations, one at/near the absorber/hole-blocking-layer, and the second at/near the absorber/electron-blocking-layer interfaces, with the former more pronounced. This ‘twin-peaks’ profile is characteristic of a p–i–n solar cell, with a layer of low-doped, high electronic quality semiconductor, between a p- and an n-layer. If the electron blocker is replaced by a gold contact, only a heterojunction at the absorber/hole-blocking interface remains. A wide variety of solar cell types exist [1] , [2] , yet in all solar cells the same basic sequence of events occurs: sunlight is absorbed in the cell’s absorber which triggers the generation, separation and transport of electronic charge carriers and their collection at opposing contacts, each selective for one of the carriers [3] , [4] . Cell types differ, however, in how this general flow chart is performed in practice, that is, in the mechanisms that make this sequence of events possible. Elucidating those mechanisms is of fundamental importance for understanding the working principle of each solar cell type, and for its further optimization. This is particularly the case when it comes to the new range of polycrystalline, organic–inorganic lead halide, perovskite cells [5] , [6] . The development of these cells has been rapid. A stream of reports has come out boasting highly efficient solid-state cells surpassing 15% efficiency [7] , [8] . Most impressive, the CH 3 NH 3 PbI 3− x Cl x cells exhibit high V OC values (~1.1 V) [5] , reaching qV OC / E Gap values of up to 0.71, a remarkably high figure for a new type of cell. In this regard, a central issue that a proposed mechanism needs to be able to explain is the source of the impressive V OC values. When a new star such as the perovskite appears in the solar cell firmament, the first question to naturally arise is: ‘How does it work?’ Here, we elucidate this question by direct measurement of electron beam-induced current (EBIC) profiles of cross-sections of CH 3 NH 3 PbI 3− x Cl x -based cells with or without a meso-structured alumina scaffold. Combining the EBIC signal with the microscope’s scanning capability, an EBIC image results, with the intensity representing the current amplitude generated in the sample. In other words, the EBIC image is a map detailing where in the cell the current is generated and at what degree of efficiency. The intensity of the peaks in the image indicates how efficient the charge separation at, cum collection from, that site in the cell is. The EBIC profile is useful for pinpointing the location of a driving force for charge separation, making it especially suited for determining the working principle of a photovoltaic device. An illustration of the EBIC experiment on a thin film device structure is shown in Fig. 1a . Here we use EBIC to study CH 3 NH 3 PbI 3− x Cl x -based photovoltaic devices, and find two peaks in EBIC intensity profile inside the absorber. This shows that the modus operandi of these devices is that of a p–i–n cell with the intrinsic absorber being of high electronic quality material. 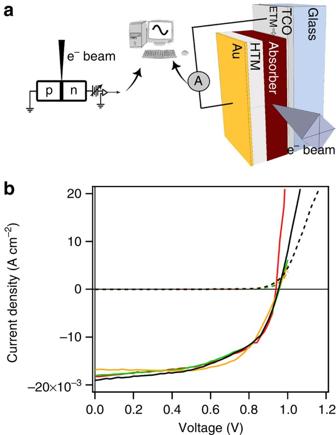Figure 1: Schematic set-up of an EBIC experiment on photovoltaic device. (a) Illustration of an EBIC experiment on a cross-section of a thin-film solar cell. The electron beam generates electron-hole pairs in the absorber material, which, after separation, creates a current generation profile inside the cell. TCO, transparent conducting oxide; HTM/ETM, hole/electron transporting material. (b)J–Vcurves of efficient devices with thick mesoporous alumina, later tested by EBIC, as described in the text. Figure 1: Schematic set-up of an EBIC experiment on photovoltaic device. ( a ) Illustration of an EBIC experiment on a cross-section of a thin-film solar cell. The electron beam generates electron-hole pairs in the absorber material, which, after separation, creates a current generation profile inside the cell. TCO, transparent conducting oxide; HTM/ETM, hole/electron transporting material. ( b ) J – V curves of efficient devices with thick mesoporous alumina, later tested by EBIC, as described in the text. Full size image Flat device with HTM Averaged photoelectrical characteristics of devices (with thick mesoporous alumina layer, taken from five devices) are: V OC =0.96 V; J SC =18.5 mA cm −2 ; fill factor=55% and a power conversion efficiency, PCE=9.9% (highest PCE=11%), which show we are in fact investigating state-of-the-art device ( Fig. 1b ). We note that devices were EBIC-investigated close to their preparation and electrical characterization time. When not investigated, devices were kept in a dark and dry environment and repeated EBIC investigations have shown similar EBIC results, therefore indicating that the cross-sections and devices were stable over the period of interest. Other devices kept in a dark desiccator have also shown stability (in comparison with the initial measurements) for more than a couple of weeks. More details about device preparation, EBIC characterization and stability are given in the Methods section. To locate where in the device most of the current is being generated, we measured the EBIC of cross-sections of a number of efficient perovskite solar cell structures. When a scanning beam of electrons, such as used in an electron microscope, is directed towards a semiconductor, it plays an analogous role to that of photons of light, generating free electrons and holes (electron-voltaic versus photovoltaic effect). Because of the high energy of the beam’s incoming electrons, multiple electron-hole pairs are generated (as high energy photons do in the case of so-called multiple exciton generation, but in much larger numbers). If a driving force for charge separation exists in the electron-excited semiconductor and contacts to collect the charge carriers are provided, an electron-voltaic cell is created, and a current is produced in the form of an EBIC signal [9] . The electron beam scans the sample, with the volume and depth of charge carrier generation determined by the voltage to which the electrons are accelerated, that is, their energy when they reach the sample surface, and by the sample’s material properties. In all the cases studied here, the absorber was the perovskite CH 3 NH 3 PbI 3− x Cl x as it readily forms larger crystallites than the other halide analogues. In Fig. 2a , a cross-sectional secondary electron (SE) image of a flat cell is shown (that is, without mp-Al 2 O 3 ; left image), with the corresponding EBIC image on the right. Two line profiles are shown in the bottom panel with the arrows indicating from which region they were taken; the colour-coding corresponds to the different layers that make up the cell. A three-dimensional (3D) surface plot of the EBIC image is shown in Fig. 1b . In the SE image, the different layers of the cell can be distinguished and are (in the direction of the arrows): the 80–100 nm Au (bright), HTM (black), perovskite absorber, 80–100 nm compact TiO 2 , ca . 700 nm F-doped tin oxide (FTO) on glass. In the EBIC line profiles, we find a ‘two-peak’ pattern, which is dominant throughout the film (regardless of HTM thickness) as can be seen in the 3D surface plot. One peak is at/near the HTM-CH 3 NH 3 PbI 3− x Cl x interface and the second peak close to the CH 3 NH 3 PbI 3− x Cl x -TiO 2 interface, with the peak closer to the HTM being consistently higher. Even though the perovskite film thickness was not uniform throughout the cross-section, an issue already addressed by others [10] , the pronounced two-peak pattern extended over the entire length of the cross-section of this cell, except where it is too thin (see below). A non-uniform region in the device showing the transition from a single EBIC peak to a double peak is shown in Supplementary Fig. 1 . The ripples on the EBIC scan in the white area to the left of the Au region in the colour-coded line profile are the background noise of the EBIC signal. The stronger EBIC background level on the right side of the sample, which is clearest in the line scans, is due to the insulating nature of the glass. 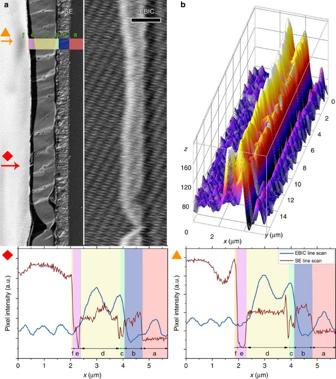Figure 2: EBIC characterization of a flat CH3NH3PbI3−xClxdevice with HTM. SE image and corresponding EBIC image of a cross-section of a solar cell without mesoporous alumina. (a) left, SE image; right, EBIC image; scale bar, 2 μm. Letters which correlate with the letters in the line scans (lower panel) designate the layers: a, glass; b, FTO; c, TiO2; d, CH3NH3PbI3−xClx; e, HTM; f, Au. (b) 3D surface plot of the EBIC image. Lower panel, line profiles of the SE and EBIC at the indicated regions: red diamond for the lower arrow and orange triangle for the higher arrow position. Overlaying colour coding as well as lettering in the graph correlates with the different layers as shown ina. Figure 2: EBIC characterization of a flat CH 3 NH 3 PbI 3− x Cl x device with HTM. SE image and corresponding EBIC image of a cross-section of a solar cell without mesoporous alumina. ( a ) left, SE image; right, EBIC image; scale bar, 2 μm. Letters which correlate with the letters in the line scans (lower panel) designate the layers: a, glass; b, FTO; c, TiO 2 ; d, CH 3 NH 3 PbI 3− x C l x ; e, HTM; f, Au. ( b ) 3D surface plot of the EBIC image. Lower panel, line profiles of the SE and EBIC at the indicated regions: red diamond for the lower arrow and orange triangle for the higher arrow position. Overlaying colour coding as well as lettering in the graph correlates with the different layers as shown in a . Full size image With an exciton binding energy of up to 50 meV [11] , and the excess energy generated by the electron beam, the generated charges in these devices are considered as free electrons and holes. These numbers were recently re-validated by reports from spectroscopic studies that have shown that also under photo-excitation, the vast majority of charges are free electrons and holes [12] . Furthermore, the experiment at hand deals with working devices that include (1) the electric fields in the device, (2) the two selective sinks for charge carriers. Both will contribute to free charge carrier population and minimize the exciton population in the measurement at hand (and in the actual working device). Variations in EBIC contrast reflect the dynamics of the carrier lifetime [9] , [13] . The intense signal close to the HTM-CH 3 NH 3 PbI 3− x Cl x interface indicates efficient hole extraction. Electrons generated there have to diffuse through the entire width of the absorber layer before being extracted at the TiO 2 interface, with increased chances of recombination the further away they are produced from their respective sink. Similar considerations apply to the holes near the TiO 2 -CH 3 NH 3 PbI 3− x Cl x interface. Combining the two decay patterns explains the decrease of the EBIC signal towards the middle of the layer and the formation of a two-peak pattern: each charge carrier is collected at a different end of the cell, forming a distinct decay pattern with its single peak, and the superposition of the hole and electron decay patterns yields a two-peak pattern. With d representing the absorber width and L n,p the electron (n) and hole (p) diffusion lengths, the junction pattern observed in the perovskite occurs only if d and L n,p are comparable (the transition from a single EBIC peak to a double peak can be seen in Supplementary Fig. 1 ). This two-peak pattern is quite distinct from other junctions. For example, a p–n junction in an absorber forms a single peak, a p–i–n structure with d >> L reveals two peaks separated by a flat region and a p–i–n structure with d << L will have but one peak of width d [14] . In a p–i–n device, a near-intrinsic (that is, low-doped) semiconductor film, which acts as solar light absorber, is contacted on both sides with p- and n-semiconductors with different work functions. These semiconductors act as the selective contacting materials. A variety of p–i–n cells exist: in the most common, amorphous Si-based one, the p- and n-semiconductors are the same as the intrinsic one, while in other cells, their materials differ from that of the intrinsic semiconductor (for example, some organic photovoltaic (OPV) cells), and energy-band offsets may exist at the p–i and i–n junctions. We note that a p–i–n model is among those models previously suggested as possible for CH 3 NH 3 PbI 3− x Cl x cells [15] , but until now, though, no experimental evidence to support this model (or another) was given. Our results do provide direct experimental evidence of the p–i–n mode of operation of a CH 3 NH 3 PbI 3− x Cl x photovoltaic device. That such a model operates in a solution-casted photovoltaic device is made all the more remarkable if we realize that the only p–i–n photovoltaic junction that is comparable with the perovskite photovoltaic junction is based on a structure that requires highly sophisticated preparation methods and high electronic quality absorber, a junction containing AlGaAs/GaAs multiple quantum wells (for comparison, amorphous hydrogenated Si, a-Si:H, has a diffusion length in the range of 0.1–0.2 μm while that of GaAs is ~1–5 μm). The high electronic quality of the absorber material is supported further by recent reports on the high charge mobility and low recombination rates [12] , [16] . The relative EBIC peak intensities are good indicators of the extraction efficiency of the two charge carriers (at the two selective interfaces). From the EBIC line scans, we calculated effective diffusion lengths, L n =1.9±0.1 μm and L p =1.5±0.2 μm ( Supplementary Fig. 2 ) [17] , [18] , [19] . These values are similar to those calculated recently by Stranks et al. [20] by modelling their time-resolved photoluminescence and absorption experimental data. The peak closer to the HTM was consistently higher than the peak closer to the TiO 2 , indicating that electrons are extracted more efficiently than holes. Our EBIC analysis of perovskite cells without an alumina scaffold revealed a two-peak signal shape characteristic of a p–i–n structure with a low-doped active layer between two selective sinks, and d ~ L . As alluded to above, a similar two-peak pattern is seen in AlGaAs/GaAs multiple quantum well p–i–n solar cells, made by molecular beam epitaxy [21] . As we will show later, this p–i–n classification of the perovskite thin-film cells also applies to perovskite cells employing mp-Al 2 O 3 as a scaffold. First though, we consider the effect of the polycrystalline nature of the perovskite material used, because transport barriers at grain boundaries can affect EBIC analyses and decrease photovoltaic performance. When we analysed the electrostatic landscape of the absorber material using scanning Kelvin probe force microscopy, we detected no significant potential variation across each grain or at its boundary ( Supplementary Fig. 3 ). This finding suggests that the grain boundaries do not contain significant depletion regions and that the electrical current is uniformly photo-generated in the bulk and at the interfaces of the grains, a situation quite different from that of CdTe but somewhat akin to that found for CIGS cells [22] , [23] . This may be the result of a low density of surface states, possibly due to the partial organic nature of this semiconductor, with the organic moieties passivating the surface (amines are well-known passivation agents for II–VI semiconductor surfaces). It is likely that such a low density of surface or interface defects also contributes to the very high V OC values obtained for these cells (because of the absence of pinning at the interfaces). Devices with a thin mp-Al 2 O 3 and HTM When we placed a thin ( ca . 100–200 nm) mp-Al 2 O 3 layer between the absorber and TiO 2 , the two-peak pattern remained ( Fig. 3 ), though the signal close to the interface with TiO 2 appeared less sharp and the peak seemed to have shifted inward, into the absorber layer. However, we believe it is plausible that the peak shift is due to a concealment effect of the electrons by the mp-Al 2 O 3 , which dilutes the current-carrying volume (the alumina does not carry any current from the electro-voltaic effect, but it does absorb some of the electrons from the e-beam), leading to the apparent peak shift. 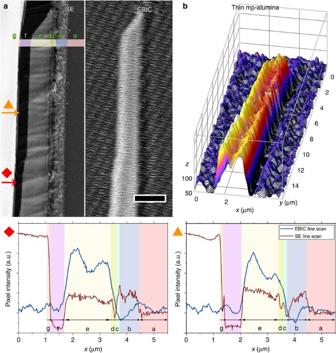Figure 3: EBIC characterization of a CH3NH3PbI3−xClxdevice with a thin mp-Al2O3and HTM. SE image and corresponding EBIC image of a cross-section of a solar cell with a thin mp-Al2O3. (a) Left, SE image; right, EBIC image; scale bar, 2 μm. Letters which correlate with the letters in the line scans (lower panel) designate the layers: a, glass; b, FTO; c, TiO2; d, mp-Al2O3; e, CH3NH3PbI3−xClx; f, HTM; g, Au. (b) 3D surface plot of the EBIC image. Lower panel, line profiles of the SE and EBIC at the indicated regions: red diamond for the lower arrow position and orange triangle for the higher arrow position. Figure 3: EBIC characterization of a CH 3 NH 3 PbI 3− x Cl x device with a thin mp-Al 2 O 3 and HTM. SE image and corresponding EBIC image of a cross-section of a solar cell with a thin mp-Al 2 O 3 . ( a ) Left, SE image; right, EBIC image; scale bar, 2 μm. Letters which correlate with the letters in the line scans (lower panel) designate the layers: a, glass; b, FTO; c, TiO 2 ; d, mp-Al 2 O 3 ; e, CH 3 NH 3 PbI 3− x Cl x ; f, HTM; g, Au. ( b ) 3D surface plot of the EBIC image. Lower panel, line profiles of the SE and EBIC at the indicated regions: red diamond for the lower arrow position and orange triangle for the higher arrow position. Full size image Devices with a thick mp-Al 2 O 3 and HTM We also examined a solar cell with a much thicker ( ca . 700 nm) mp-alumina scaffold. In Fig. 4 , the SE and EBIC images of a cross-section of this cell are shown. From the 3D surface plot of the EBIC image ( Fig. 4b ), we find there is still a peak in the absorber close to the HTM, more dominant than the peaks we observed close to the HTM before ( Figs 2 and 3 ). 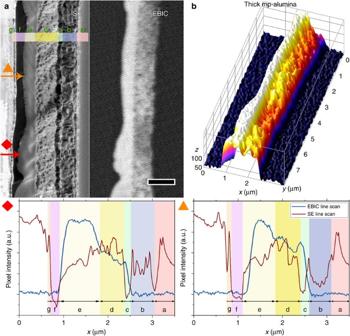Figure 4: EBIC characterization of a CH3NH3PbI3−xClxdevice with a thick mp-Al2O3and HTM. SE image and corresponding EBIC image of a cross-section of a solar cell with a 700 nm thick mp-Al2O3. (a) left, SE image; right, EBIC image; scale bar, 1 μm. Letters which correlate with the letters in the line scans (lower panel) designate the layers: a, glass; b, FTO; c, TiO2; d, mp-Al2O3; e, CH3NH3PbI3−xClx; f, HTM; g, Au. (b) 3D surface plot of the EBIC image. Lower panel, line profiles of the SE and EBIC at the indicated regions: red diamond for the lower arrow position and orange triangle for the higher arrow position. Figure 4: EBIC characterization of a CH 3 NH 3 PbI 3− x Cl x device with a thick mp-Al 2 O 3 and HTM. SE image and corresponding EBIC image of a cross-section of a solar cell with a 700 nm thick mp-Al 2 O 3 . ( a ) left, SE image; right, EBIC image; scale bar, 1 μm. Letters which correlate with the letters in the line scans (lower panel) designate the layers: a, glass; b, FTO; c, TiO 2 ; d, mp-Al 2 O 3 ; e, CH 3 NH 3 PbI 3− x Cl x ; f, HTM; g, Au. ( b ) 3D surface plot of the EBIC image. Lower panel, line profiles of the SE and EBIC at the indicated regions: red diamond for the lower arrow position and orange triangle for the higher arrow position. Full size image However, the EBIC peak usually located close to the TiO 2 interface is now almost entirely obscured by the alumina, although remnants of the signal can still be detected. Furthermore, we note that in areas that do not have a capping layer of absorber on top of the mp-Al 2 O 3 , we do not see an EBIC signal (or a very faint one; see Supplementary Fig. 4 ), implying that this cell does not operate as a nanocomposite, a so-called bulk heterojunction as was speculated before [5] , that is to say that the inner mixing of absorber and HTM in the pores are not significant for the functioning of the device per se , and the mixing with mp-Al 2 O 3 likely functions to improve surface coverage. These are indications that the p–i–n model of the cell still holds regardless of the mp-alumina. Furthermore, it suggests that a possible path to improve these cells is to improve the uniformity of the perovskite coverage, a feature that is, to a limited extent, obtained with the alumina scaffold [7] , [10] . In terms of device operation, this inhomogeneity can be visualized as (photo-)diodes with different V OC s connected in parallel, therefore reducing the cell’s overall V OC . The effect on V OC stems from the different dark current that each diode will have [24] , [25] . The local absorber thickness may also affect the local J SC . Devices with a thin mp-Al 2 O 3 and without HTM Finally, in Fig. 5 , we look at a structure without HTM (a thin mp-Al 2 O 3 was used to prevent shunts from the Au back contact to the TiO 2 ). 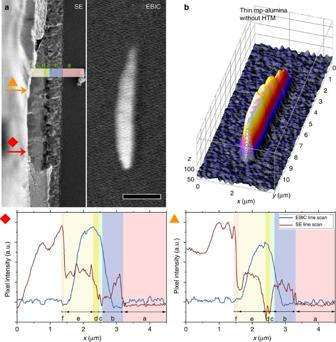Figure 5: EBIC characterization of a CH3NH3PbI3−xClxdevice with a thin mp-Al2O3without HTM. SE image and corresponding EBIC image of a cross-section of a solar cell with a thin mp-Al2O3and without HTM. (a) left, SE image; right, EBIC image; scale bar, 2 μm. Letters which correlate with the letters in the line scans (lower panel) designate the layers: a, glass; b, FTO; c, TiO2; d, mp-Al2O3; e, CH3NH3PbI3−xClx; f, Au. (b) 3D surface plot of the EBIC image. Lower panel, line profiles of the SE and EBIC at the indicated regions: red diamond for the lower arrow position and orange triangle for the higher arrow position. Figure 5: EBIC characterization of a CH 3 NH 3 PbI 3− x Cl x device with a thin mp-Al 2 O 3 without HTM. SE image and corresponding EBIC image of a cross-section of a solar cell with a thin mp-Al 2 O 3 and without HTM. ( a ) left, SE image; right, EBIC image; scale bar, 2 μm. Letters which correlate with the letters in the line scans (lower panel) designate the layers: a, glass; b, FTO; c, TiO 2 ; d, mp-Al 2 O 3 ; e, CH 3 NH 3 PbI 3− x Cl x ; f, Au. ( b ) 3D surface plot of the EBIC image. Lower panel, line profiles of the SE and EBIC at the indicated regions: red diamond for the lower arrow position and orange triangle for the higher arrow position. Full size image Here, we could not detect a two-peak pattern, only a single, broad peak, with its maximum intensity close to the TiO 2 and a slow decrease of the signal towards the Au back contact. The absorber thickness in the region between the two arrows is ca . 1 μm, comparable to the thickness of the absorber in Fig. 3 ( ca . 1.3 μm at the thin region). The slow decrease in the EBIC signal towards the Au back contact indicates there is no (or very little) band bending from a Schottky junction at the Au-absorber interface. We therefore conclude that in the absence of a hole-transporting material, the cell functions as a heterojunction between the absorber and the TiO 2 , with the area of maximum current production and, thus, the position of the junction centre in the perovskite located close to the TiO 2 . This structure suggests the possibility of increasing the voltage by driving the perovskite into strong inversion. We conclude that these cells, both in the thin film and in the inert mesoporous configuration, operate as a p–i–n device with a high electronic quality -i- layer, and where the quasi-Fermi levels split within this said layer. This is in contrast with other devices, such as p–n junctions where the quasi-Fermi level splitting can take place also outside the space charge region, in the so-called selective contacts. The high V OC arises from having two (half-) junctions in series, each being a separate hetero-junction that contributes to minimize the dark current and maximize the photocurrent, and by their mutual contribution lead to an increased V OC (ref. 26 ). This is summarized in the schematic band diagram of a p–n junction ( Fig. 6a ), an ‘a-Si:H’-like p–i–n junction ( Fig. 6b ), and our suggested p–i–n band diagram for CH 3 NH 3 PbI 3− x Cl x perovskite-based cells ( Fig. 6c ), emphasizing the in-homogeneous built-in field in this device in comparison to other p–i–n devices. 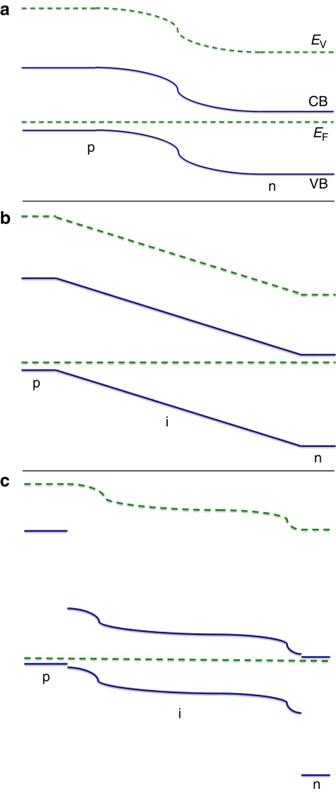Figure 6: A schematic band diagram of common photovoltaic devices. (a) a p–n junction solar cell. (b) A p–i–n solar cell with homogenous built-in electric field (‘a-Si:H’-like). (c) CH3NH3PbI3−xClxperovskite-based cells. The diagrams are not to scale and show only relative positions of the energy bands. Figure 6: A schematic band diagram of common photovoltaic devices. ( a ) a p–n junction solar cell. ( b ) A p–i–n solar cell with homogenous built-in electric field (‘a-Si:H’-like). ( c ) CH 3 NH 3 PbI 3− x Cl x perovskite-based cells. The diagrams are not to scale and show only relative positions of the energy bands. Full size image The data show that the electron extraction efficiency is somewhat higher than that of holes, and we estimate the effective diffusion lengths for both charge carriers to be greater than 1 μm. Similar to the efficient CIGS cells, the perovskite absorbers are composed of oriented high-quality crystalline grains [5] , [20] with benign grain boundaries and a low density of surface/interface states. This explains the high efficiency and high qV OC / E gap ratio in the CH 3 NH 3 PbI 3− x Cl x perovskite-based cells. In the absence of an HTM, we find little or no field at the perovskite/Au junction and the active junction is then between the perovskite and the TiO 2 . Device fabrication FTO transparent conducting substrates (Pilkington TEC15) were cut and cleaned by sequential 15 min sonication in warm aqueous alconox solution, deionized water, acetone and ethanol, followed by drying in a N 2 stream. A compact ca . 100 nm thin TiO 2 was then applied to the clean substrate by spray pyrolysis of 200 mM titanium diisopropoxide bis(acetylacetonate) solution in isopropanol using air as carrier gas on a hot plate set to 350 °C, followed by annealing at 500 °C for 1 h in air. A mp-Al 2 O 3 scaffold was prepared by spin-coating an alumina nanoparticle paste ( d =50 nm) on the compact titania-coated substrates. An alumina nanoparticle suspension in water was used as the basis for the alumina paste. First, the water was replaced by ethanol via repeat separation and re-suspension in ethanol to obtain a 10%wt suspension. Ten grams of this suspension were mixed with 8.33 g of ethyl cellulose solution (5 g of ethanol, 3.33 g α-terpineol, 1 g of 10 cP ethyl cellulose and 1 g of 46 cP ethyl cellulose). The ethanol was removed completely by a rotary evaporator before re-dispersing the paste with ethanol by adding ethanol 2.5 times the weight of the paste. The paste was spin-coated at 500 r.p.m. (4.2 g force) for 5 s, followed by 3,000 r.p.m. (151 g force) for 45 s and then sintered at 550 °C for 2 h to give a ca . 700 nm thin porous film. This basic paste was diluted with ethanol prior to use in a 1:1 weight ratio to form the thin alumina film. A CH 3 NH 3 PbI 2 Cl solution was prepared as described elsewhere [21] . In short, CH 3 NH 3 I was prepared by mixing methyl amine (40% in methanol) with hydroiodic acid (57% in water; caution: exothermic reaction) in a 1:1 molar ratio in a 100 ml flask under continuous stirring at 0 °C for 2 h. CH 3 NH 3 I was then crystallized by removing the solvent in a rotary evaporator, washing three times in diethyl ether for 30 min and filtering the precipitate. The material, in the form of white crystals, was then dried overnight in vacuum at 60 °C. It was then kept in a dark, dry environment until further use. A 40%wt solution of CH 3 NH 3 PbI 3− x Cl x was prepared by mixing PbCl 2 and CH 3 NH 3 I in a 1:3 molar ratio in N′N-dimethylformamide and heating it to 60 °C until a clear yellow solution was formed. To coat the substrate, the solution was spin-coated in two stages: 5 s at 500 r.p.m. and then at 1,500 r.p.m. (38 g force) for 30 s. The substrate was then heated on a hot plate set at 100 °C for 45 min, after which the substrate turned deep dark brown in colour. To finish the device fabrication, a 100 μl hole conductor solution (84 mg spiro-MeOTAD in 1 ml chlorobenzene, mixed with 7 μl of tert-butylpyridine and 15 μl of 170 mg/ml LiTFSI, bis(trifluoromethane)sulphonamide, in acetonitrile), was applied by spin-coating 5 s at 500 r.p.m., then at 1,500 r.p.m. for 30 s, and then 100 nm gold contacts were thermally evaporated on the back through a shadow mask with 0.24 cm 2 rectangular holes. Device characterization The J – V characteristics were measured with a Keithley 2400-LV SourceMeter and controlled with a Labview-based, in-house designed program. A solar simulator (ScienceTech SF-150) equipped with a 1.5AM filter and calibrated with a Si solar cell IXOLAR High Efficiency SolarBIT (IXYS XOB17-04 × 3) was used for illumination. The devices were characterized through a 0.16 cm 2 mask. EBIC measurements After characterizing the devices in the solar simulator, the samples were cleaved by hand after scribing the glass on the back and immediately loaded into the scanning electron microscope vacuum chamber for EBIC measurements. Scanning electron microscope images were taken on a Zeiss SUPRA high-resolution microscope equipped with a Specimen Current Amplifier (GW electronics Inc., Type 31). The gold back contact was connected to the sample holder and, through it, to the preamplifier by a small micromanipulator to enable measuring the sample current. Using the Grün formula, we calculated a penetration depth of ca . 20 nm under working conditions [9] (1.5 keV; working distance of ca . 5 mm and density of the perovskite taken as ca . 4 g ml −1 (ref. 16 ), suggesting a lateral EBIC resolution of the same order of magnitude. Images were processed using the Fiji package of ImageJ 1.48. A word of caution: even the relatively low energy, 1.5 keV, electron beam damages the sample over time, with increased exposure. Supplementary Fig. 5 shows the decrease in EBIC intensity with sequential scans. A clear deterioration of the EBIC signal is observed after several acquisition scans. How to cite this article: Edri, E. et al. Elucidating the charge carrier separation and working mechanism of CH 3 NH 3 PbI 3− x Cl x perovskite solar cells. Nat. Commun. 5:3461 doi: 10.1038/ncomms4461 (2014).